A gatekeeper helix determines the substrate specificity of Sjögren–Larsson Syndrome enzyme fatty aldehyde dehydrogenase Mutations in the gene coding for membrane-bound fatty aldehyde dehydrogenase (FALDH) lead to toxic accumulation of lipid species and development of the Sjögren–Larsson Syndrome (SLS), a rare disorder characterized by skin defects and mental retardation. Here, we present the crystallographic structure of human FALDH, the first model of a membrane-associated aldehyde dehydrogenase. The dimeric FALDH displays a previously unrecognized element in its C-terminal region, a ‘gatekeeper’ helix, which extends over the adjacent subunit, controlling the access to the substrate cavity and helping orientate both substrate cavities towards the membrane surface for efficient substrate transit between membranes and catalytic site. Activity assays demonstrate that the gatekeeper helix is important for directing the substrate specificity of FALDH towards long-chain fatty aldehydes. The gatekeeper feature is conserved across membrane-associated aldehyde dehydrogenases. Finally, we provide insight into the previously elusive molecular basis of SLS-causing mutations. Free aldehydes are toxic to cells due to their high reactivity with free amino groups of macromolecules such as proteins and lipids. Cells protect themselves by rapid conversion of free aldehydes into non-toxic fatty acids by aldehyde dehydrogenases (ALDHs) [1] . Long-chain aliphatic aldehydes are generated at cellular membranes as a consequence of lipid metabolism and oxidative stress-associated lipid peroxidation [2] . These aldehydes are not accessible by cytosolic ALDHs and are processed by specific membrane-associated ALDH. In addition to their detoxifying function, these enzymes play a major role in redirecting these energy-rich metabolites into salvage pathways for lipid biosynthesis [3] . In humans, the ALDH3A2 gene encodes a specific membrane-bound fatty aldehyde dehydrogenase (FALDH, E.C. 1.2.1.48), which is responsible for the conversion of long-chain fatty aldehydes into their corresponding fatty acids [3] . The disruption of FALDH function results in a severe metabolic disorder, the Sjögren–Larsson Syndrome (SLS, MIM 270200) (ref. 4 ). The pathology of this autosomal recessive disease manifests with symptoms such as ichtyosis, spasticity and mental retardation [5] . FALDH plays an important detoxifying role in different lipid degrading pathways ( Fig. 1 ). This includes the enzymatic degradation of sphingosine-1-phosphate, which is a ligand for five specific G protein-coupled receptors [6] , implicating sphingosine-1-phosphate into a series of cellular processes such as proliferation, growth, movement, survival and immunity [7] . Impaired FALDH function in CHO-K1 cells results in an abnormal sphingosine-1-phosphate metabolism [3] . FALDH also clears the products of ether lipids degradation such as platelet-activating factor and plasmalogens [8] , molecules that are used for inter and intracellular signalling [9] , [10] , [11] , [12] . In addition, FALDH has been shown to protect cells against oxidative stress-induced lipid peroxidation [2] and its expression is regulated by proliferator-activated receptor alpha [13] . 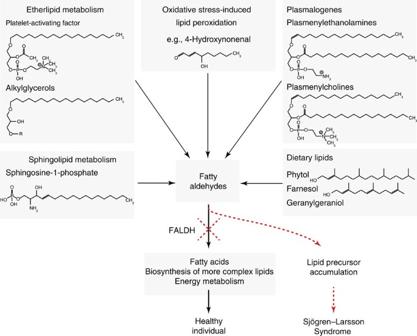Figure 1: Role of FALDH in selected membrane lipid metabolic pathways. In cells, fatty aldehydes are produced during oxidative stress-induced lipid peroxidation2and by enzymatic degradation of a series of lipids including sphingosine-1-phosphate3, plasmalogens8and alkylglycerols such as the platelet-activating factor12. Impaired FALDH function has been shown to alter the metabolic profiles of connected pathways and can lead to the development of the SLS (red arrows)3,22. Figure 1: Role of FALDH in selected membrane lipid metabolic pathways. In cells, fatty aldehydes are produced during oxidative stress-induced lipid peroxidation [2] and by enzymatic degradation of a series of lipids including sphingosine-1-phosphate [3] , plasmalogens [8] and alkylglycerols such as the platelet-activating factor [12] . Impaired FALDH function has been shown to alter the metabolic profiles of connected pathways and can lead to the development of the SLS (red arrows) [3] , [22] . Full size image FALDH belongs to the superfamily of ALDHs, which are homo-oligomeric enzymes characterized by the presence of a cofactor-binding domain, a catalytic domain and a bridging domain involved in oligomerization [14] . Depending on the alternatively spliced hydrophobic carboxy-terminal (C-terminal) transmembrane domain, FALDH is anchored into the membranes of the endoplasmic reticulum or peroxisomes, respectively [15] . A deep funnel-like structure formed at the interface between catalytic- and cofactor-binding domain gives access to the catalytic cysteine (Cys-241 in human FALDH) [14] . The amino acids lying in the funnel have been proposed to be involved in substrate selectivity [14] , [16] . In addition, FALDH has two distinctive hydrophobic domains at the C terminus, one of which is predicted to form a transmembrane helix that anchors the protein to the lipidic bilayer [17] . So far, only limited information on the FALDH structure and function is available, presumably because this membrane-bound enzyme is challenging to work with. We have previously demonstrated that the native active form of FALDH is a homodimer [18] . On the basis of homology modelling using the soluble ALDH3A1 enzyme (66% sequence identity with FALDH), Lloyd et al . [14] , [19] have proposed a unique reaction mechanism for FALDH that differs from other ALDHs. A series of ALDHs have been shown to bind NAD in a conformation that results in a pro- R -specific hydride transfer during catalysis [20] . For ALDH3A1, an alternative NAD-binding mode has been reported, pointing towards a pro- S stereoselectivity [14] . However, a recently published structure shows ALDH3A1 binding NAD in a clear pro- R -specific manner [21] . A key unresolved question in the function of FALDH enzymes is how substrate specificity is achieved. Long-chain aldehydes are specifically metabolized by this enzyme. Therefore, a loss-of-function for FALDH is barely compensated by other ALDHs, even by those that have a high degree of sequence similarity [22] . In this study, we present the crystallographic structure of human FALDH, which represents the first structure of a membrane-specific aldehyde dehydrogenase. This study reveals a novel structural element, represented by a C-terminal hydrophobic helix that is required for efficient oxidation of long-chain fatty aldehydes. This helix, located at the interface between the membrane and the entry to the substrate tunnel, is conserved in other membrane-associated aldehyde dehydrogenases. Structural modelling and mutational studies indicate that this structural feature is critical for the selectivity and transfer of substrates and products from and to the lipid bilayer. Thus, the FALDH structure provides a powerful novel basis to examine the molecular mechanism of mutations causing the SLS. Human FALDH forms a symmetrical dimer Human FALDH cDNA was cloned into a Strep-tag fusion vector, expressed in E.coli and subsequently purified by affinity chromatography and gel filtration. Purified FALDH was assayed for crystallization; yielding three-dimensional crystals, which were used for X-ray diffraction experiments (see Methods). FALDH crystals containing amino acids 1–460 belong to the space group P 212121 and diffracted up to a resolution of 2.1 Å. Initial phases were obtained by molecular replacement using the human class 3 aldehyde dehydrogenase ALDH3A1 (3SZA [16] ) as search model. The final model contains two chains of FALDH in the asymmetric unit and was refined to an Rwork of 19.96% and an Rfree of 22.26% (see Table 1 ). All amino acids present in the expression construct, including amino acid 1–460 of the human FALDH sequence, were modelled for Chain A. Conversely, in chain B, the residues 458–460 showed weak electron density, indicating that they are not well-ordered and hence were not included in the model. For an illustration of a typical electron density map, see Supplementary Fig. 1 . Both subunits adopt very similar symmetrical, homodimeric structure and conformations (r.m.s.d. overall atoms=0.212 Å) ( Fig. 2 ). Table 1 Data collection and refinement statistics. 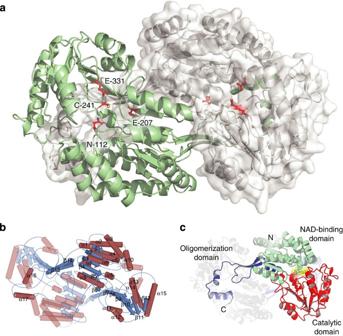Figure 2: Structure of human FALDH. (a) FALDH is a symmetrical homodimer with a large dimerization interface. One subunit is shown in cartoon representations (green), the other as surface model (grey). Each dimer exhibits two active sites (catalytic side chains are shown in red). (b) The FALDH secondary structure (blue, β-sheets; red, α-helices): a central plane of beta sheets (β1–5 of each dimer) and two staggered, spiral-like alignment (β 6–14) that are enveloped by alpha helices (α 1–15). α16+17 are arranged around the substrate entry funnel of the respective other momomer. (c) The domain structure of FALDH includes a NAD-binding domain (green residues 1–79 and 103–208), a catalytic domain (red residues 209–419) and a C-terminal oligomerization domain (blue residues 82–102 and 420–443). Full size table Figure 2: Structure of human FALDH. ( a ) FALDH is a symmetrical homodimer with a large dimerization interface. One subunit is shown in cartoon representations (green), the other as surface model (grey). Each dimer exhibits two active sites (catalytic side chains are shown in red). ( b ) The FALDH secondary structure (blue, β-sheets; red, α-helices): a central plane of beta sheets (β1–5 of each dimer) and two staggered, spiral-like alignment (β 6–14) that are enveloped by alpha helices (α 1–15). α16+17 are arranged around the substrate entry funnel of the respective other momomer. ( c ) The domain structure of FALDH includes a NAD-binding domain (green residues 1–79 and 103–208), a catalytic domain (red residues 209–419) and a C-terminal oligomerization domain (blue residues 82–102 and 420–443). Full size image Each FALDH subunit in the asymmetric unit adopts the canonical aldehyde dehydrogenase fold, including an amino-terminal (N-terminal) cofactor-binding domain (residues 1–79 and 103–208), a catalytic domain (residues 209–419) and an oligomerization domain (residues 82–102 and 420–443) that connects the two subunits of the dimer ( Fig. 2c ). The C-terminal residues 445–460 form an alpha helix that is not present in any of the known structures of soluble ALDHs (see below). In the natural FALDH sequence, this region is directly followed by a predicted transmembrane alpha-helical region (residues 464–485) that was not included in the expression constructs, due to incompatibility with the protein production process. The truncated and full-length form of FALDH exhibited comparable specific activities. The catalytic and cofactor-binding domains of human FALDH (huFALDH) are structurally similar to that of cytosolic rat and human ALDH3A1 (with r.m.s.d. of 0.718 and 0.543, respectively) and contain all the structural features that characterize the ALDH family [14] , [16] , [20] . The catalytic domain contains the catalytic cysteine (Cys-241, corresponding to Cys-302 in mammalian class 1 and class 2 ALDHs [16] ), which is located in a deep cleft between the two domains ( Fig. 2 ). The cofactor and the substrate access the catalytic site from opposite sides. While Cys-241 is readily accessible from the cofactor site, substrates access the catalytic site through a deep funnel with an approximate length of 25 Å ( Fig. 3 ). The cofactor-binding site is highly conserved in the superfamily of ALDHs ( Supplementary Fig. 2 ). In the present structure, residues Ile-108, Trp-111, Asn-112, Glu-138, Ser-140, Val-167, Thr-170, Leu-174, Gly-185, Val-189, Ile-192, Val-193, Trp-231 and Phe-333 are expected to be involved in either hydrogen bonds or van der Waals contacts with the NAD cofactor. All of these residues are conserved between rat ALDH3a1 (1ad3 (ref. 14 )) and FALDH. 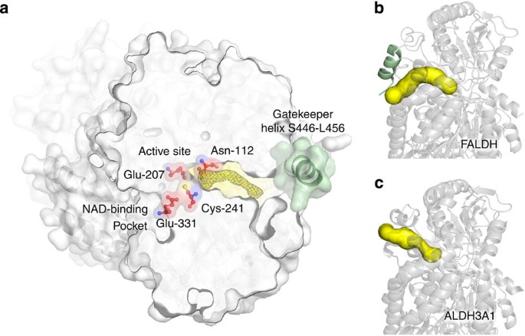Figure 3: An additional gatekeeper helix constrains substrate specificity by restricting the substrate binding funnel. (a) Cross section through the active site of FALDH. The NAD-binding pocket and the substrate funnel positioned on opposite sides of the enzyme and merge in its central active site. Active site residues are indicated in red (Asn-112, Glu-207, Cys-241 and Glu-331). The electron density found in the substrate funnel is indicated in yellow. The electron density mesh was generated at 1.2 sigma within 1.6 Å around a hexadecanoic acid molecule, which was previously modelled into the electron density. The gatekeeper helix, covering the substrate funnel entrance is shown in green. The substrate funnels of (b) FALDH and (c) ALDH3A1 (3sza) were characterized using the MOLE toolkit for PyMOL. While in FALDH, the additional gatekeeper helix (shown in green) creates a kink in the channel (shown in yellow), the wide, linear arrangement of the substrate funnel entrance of ALDH3A1 is not restricted. Figure 3: An additional gatekeeper helix constrains substrate specificity by restricting the substrate binding funnel. ( a ) Cross section through the active site of FALDH. The NAD-binding pocket and the substrate funnel positioned on opposite sides of the enzyme and merge in its central active site. Active site residues are indicated in red (Asn-112, Glu-207, Cys-241 and Glu-331). The electron density found in the substrate funnel is indicated in yellow. The electron density mesh was generated at 1.2 sigma within 1.6 Å around a hexadecanoic acid molecule, which was previously modelled into the electron density. The gatekeeper helix, covering the substrate funnel entrance is shown in green. The substrate funnels of ( b ) FALDH and ( c ) ALDH3A1 (3sza) were characterized using the MOLE toolkit for PyMOL. While in FALDH, the additional gatekeeper helix (shown in green) creates a kink in the channel (shown in yellow), the wide, linear arrangement of the substrate funnel entrance of ALDH3A1 is not restricted. Full size image The substrate funnel entrance, on the opposite side of the cofactor-binding site, is built up by residues Ser-58, Gln-59, Ile-62, Thr-63, Gly-66, Glu-67, Asp-69, Phe-70, Glu-73, Lys-85, Asn-87, Val-88, Leu-89, Asn-112, Tyr-113, Val-116, Leu-117, Gln-120, Trp-231, Met-235, Thr-240, Cys-241, Ile-242, Ile-389, Met-390, Phe-392, Thr-293, Asn-395 Phe-399, His-411, Phe-454, Leu-455 and Lys-457. While the cofactor-binding site is highly conserved, only 13 of the 33 amino acids building up the substrate funnel are conserved between FALDH and rat liver ALDH3A1, which could explain in part the difference in substrate specificity [14] , [16] . FALDH was crystallized in the absence of a ligand; however, a tetrahedron-shaped electron density peak was found at the catalytic site at an approximate distance of 4.5 Å from the thiol group of the catalytic Cys-241 residue. This peak is connected to a slightly weaker electron density area of tubular shape and that extends through most of the substrate tunnel cavity (yellow density map, Fig. 3a ). This suggests the presence of a molecule formed by a long and potentially flexible chain, with an electron-rich head group at the substrate site. Mass spectrometric analysis of a lipid extract obtained from our purified FALDH samples indicated the presence of a 0.8:1 mixture of hexadecanoic and octadecanoic acid ( Supplementary Fig. 3 ). These compounds are also the natural products of FALDH. Their presence in our protein extracts could result from co-purification from E.coli cells that contain these metabolites in their membranes. We would however like to state that the electron density was not sufficiently well-defined to identify the molecules conclusively. Therefore, an occupation of the substrate funnel, for example, by the CHES buffer ( N -Cyclohexyl-2-aminoethanesulfonic acid) used for protein crystallization (although the CHES structure does not entirely match the shape of the observed electron density) or analogue molecules is possible. The FALDH reaction mechanism The reaction mechanism for FALDH has been proposed to be based on a nucleophilic attack of the fatty aldehyde substrate by Cys-241. Lloyd et al . [19] speculate that the resultant thiohemiacetal is deprotonated by Tyr-410, which initiates a hydride transfer from the substrate to the NAD cofactor. Glu-207 would then mediate a nucleophilic attack of a hydroxide anion, and the fatty acid product is eventually released ( Fig. 4a ). To investigate the effect of the FALDH reaction mechanism on substrate specificity, we performed site-directed mutagenesis of residues involved in catalysis (C241S, E207Q and Y410F). An additional set of conserved residues was selected based on their proximity to the active site in the crystal structure, or was selected based on published evidence for their catalytic function in other ALDH isozymes (E331Q, N112A and Y113F). Mutant FALDH variants were cloned, purified and their correct folding was verified by circular dichroism measurements. A fluorometric assay was used to determine the enzymatic activity of purified wild-type and mutated FALDH proteins (see Methods). Three medium to long aliphatic chain fatty aldehydes, octadecanal, dodecanal and hexadecanal were used as substrates. Improper recycling of hexadecanal derived from sphingosine-1-phosphate catabolism and other fatty aldehydes originating from other sources has been proposed to be a major cause for SLS [3] . Enzymatic assays demonstrated that, as expected, Cys-241 and Glu-207 play a critical role in catalysis, since the corresponding mutants showed no activity against any of the substrates ( Fig. 4b ). The Y410F mutant showed normal V max / K M levels against octanal and dodecanal and a somewhat reduced but still considerable catalytic capacity for hexadecanal. Hence, Tyr-410 is not essential for FALDH activity, but may be required for efficient substrate turnover. The enzymatic assays also revealed important roles for Glu-331 and Asn-112: proteins mutant for E331Q and N112A did not exhibit enzymatic activity in our assay. In contrast, mutating Tyr-113 had no effect on catalysis ( Fig. 4b ). 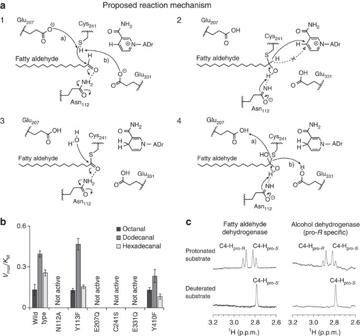Figure 4: A proposed reaction mechanism for FALDH. (a) Reaction schemes for the oxidation of long-chain fatty aldehydes by FALDH. (1) Cys-241 is activated by a general base (possible active residues are (a) Glu-207 or (b) Glu-331), and then initiates a nucleophilic attack on the carbonyl carbon of the aldehyde. Correct positioning of the polar aldehyde head group is supported by Asn-112. (2) The formed oxyanion collapses, eliminating a hydride ion, which is transferred to NAD. (3) A proton is abstracted from a water molecule, which initiates a nucleophilic attack on the carbonyl carbon of the covalently bound substrate. (4) A recurrent oxyanion collapse terminates the thiohemiacetal bond and releases the fatty acid product. (b) Influence of mutated active site residues on enzymatic capacity. Mutations where introduced by site-directed mutagenesis and correct folding of the purified enzymes was verified (see Methods). N112A, E207Q, C241S and E331Q mutations completely abolished all measurable enzymatic activity. Y113F had now significant effect on enzymatic activity. Exchanging the previously reported catalytic amino acid Y410 with phenylalanine had only small impact on the FALDH reaction. Data are shown as mean±s.e.m. (calculated with error propagation,n=3). (c) Stereoselectivity of the FALDH reaction:1H NMR spectroscopy was used to monitor the stereospecific collapse of the NAD C4-H splitting pattern (C4-Hpro-S: 2.77; C4-Hpro-R: 2.87 p.p.m.) during the enzymatic hydride transfer from deuterated substrates to the cofactor (spectra after 60 min of reaction time are shown). As control, we used the pro-R-specific horse liver alcohol dehydrogenase and 1,2-[D]-ethanol. For the closely related ALDH3A1, a special NAD-binding mode with a presumed pro-Sstereoselectivity was reported. In contrast, for FALDH, we exclusively observe the presence of the downfield C4-Hpro-Ssignal (2.77 p.p.m.), indicating a specific deuteration of the pro-Rposition. Additional controls for this experiment are depicted inSupplementary Fig. 4b. Figure 4: A proposed reaction mechanism for FALDH. ( a ) Reaction schemes for the oxidation of long-chain fatty aldehydes by FALDH. (1) Cys-241 is activated by a general base (possible active residues are (a) Glu-207 or (b) Glu-331), and then initiates a nucleophilic attack on the carbonyl carbon of the aldehyde. Correct positioning of the polar aldehyde head group is supported by Asn-112. (2) The formed oxyanion collapses, eliminating a hydride ion, which is transferred to NAD. (3) A proton is abstracted from a water molecule, which initiates a nucleophilic attack on the carbonyl carbon of the covalently bound substrate. (4) A recurrent oxyanion collapse terminates the thiohemiacetal bond and releases the fatty acid product. ( b ) Influence of mutated active site residues on enzymatic capacity. Mutations where introduced by site-directed mutagenesis and correct folding of the purified enzymes was verified (see Methods). N112A, E207Q, C241S and E331Q mutations completely abolished all measurable enzymatic activity. Y113F had now significant effect on enzymatic activity. Exchanging the previously reported catalytic amino acid Y410 with phenylalanine had only small impact on the FALDH reaction. Data are shown as mean±s.e.m. (calculated with error propagation, n =3). ( c ) Stereoselectivity of the FALDH reaction: 1 H NMR spectroscopy was used to monitor the stereospecific collapse of the NAD C4-H splitting pattern (C4-H pro- S : 2.77; C4-H pro- R : 2.87 p.p.m.) during the enzymatic hydride transfer from deuterated substrates to the cofactor (spectra after 60 min of reaction time are shown). As control, we used the pro- R -specific horse liver alcohol dehydrogenase and 1,2-[D]-ethanol. For the closely related ALDH3A1, a special NAD-binding mode with a presumed pro- S stereoselectivity was reported. In contrast, for FALDH, we exclusively observe the presence of the downfield C4-H pro- S signal (2.77 p.p.m. ), indicating a specific deuteration of the pro- R position. Additional controls for this experiment are depicted in Supplementary Fig. 4b . Full size image Next, we performed 1 H NMR measurements with deuterated aldehydes, to investigate the stereospecificity of the hydride transfer in purified FALDH (substrate:[1- 2 D]-hexadecanal). The two diastereotopic C4 protons of NADH can be distinguished by their distinct chemical shift signature. The pro- S proton faces the adenine ring of NADH and is thus shielded via a ring current effect resulting in an upfield chemical shift compared with the pro- R proton [23] , [24] , [25] , [26] . Enzymatic deuteration of NAD leads to an R - or S -specific collapse of the corresponding NMR splitting pattern [23] , [27] . Comparison of FALDH with a horse liver alcohol dehydrogenase control (substrate: [1,2- 2 D]-ethanol) with known pro- R stereoselectivity [28] indicated that the hydride transfer in FALDH is clearly pro- R specific ( Fig. 4c ). This result was corroborated by monitoring the direct hydride transfer by mass spectrometry ( Supplementary Fig. 4a ). Compared with 1 H chemical shift literature values, the NADH signals observed in the respective 2–3 p.p.m. region are shifted upfield (2.77/2.87 versus 2.67/2.77 p.p.m.) (refs 24 , 25 ). Control experiments showed that this shift can be explained by the different measurement temperature (37 °C compared with 25 °C that was used in earlier NMR experiments, Supplementary Fig. 4b ). In addition, a conformational analysis confirmed the identity of the C4 pro- S proton, which should display a greater splitting due to scalar coupling to the C5 proton (for example, 3J(C5-H pro- S )=2.59 Hz for sample 5 at 25 °C, Supplementary Fig. 4b ) [25] . These findings suggest an alternative model for the reaction mechanism of FALDH (see Fig. 4a ) than reported earlier [19] ( Supplementary Fig. 4c ). The first step involves the activation of the catalytic Cys-241 by deprotonation and subsequent substrate binding ( Fig. 4a (1). For other ALDHs it has been debated, whether the general base responsible for activation of Cys-241 is the equivalent to Glu-207 (refs 29 , 30 , 31 , 32 , 33 ) or Glu-331 (refs 34 , 35 , 36 ) in FALDH (both scenarios are indicated in Fig. 4a by (a) and (b) respectively). It has been shown that Glu-331 interacts with the ribose-backbone of NAD and assists correct cofactor binding and orientation [20] , [26] , [37] , [38] . Once Cys-241 is deprotonated, it performs a nucleophilic attack on the carbonyl carbon of the fatty aldehyde, which forms a thiohemiacetal [39] , [40] , [41] . Asn-112 supports the orientation of the polar head group by coordinating to the substrate oxygen (shown in dashed line) and subsequently stabilizes a tetrahedral reaction intermediate [20] , [34] . In a second step, ( Fig. 4a (2)) the collapse of the primarily formed oxyanion then initiates a hydride transfer to the NAD cofactor in a pro- R manner, as discussed above. Subsequently, a water molecule is deprotonated by Glu-207 or Glu-331 and triggers a nucleophilic attack of the hydroxide anion on the carbonyl carbon of the ( Fig. 4a (3) (refs 32 , 33 , 34 ). In a final step ( Fig. 4a (4)), a repeated collapse of the oxyanion forms the fatty acid product and releases the covalent bond to Cys-241, which remains activated or can be potentially reactivated. With the here presented structure, unequivocal assignment of the functions of Glu-207/331 is not feasible. However, the activity assays indicate that both residues play an important role and that the loss of one of them cannot be compensated by the function of the other ( Fig. 4b ). The distance of Cys-241 to Glu-331 is 2.9 Å, with several water molecules in proximity that potentially can mediate the deprotonation of Cys-241. Glu-207 is pointing away from Cys-207 with a distance of 7.7 Å. Similar orientations and distances have also been found in other ALDHs [20] , [34] . However, this may not reflect the actual position during catalysis, since a high flexibility of a catalytically active Glu-207 equivalent has been reported [30] , [31] , [32] . Although the specific catalytic role of Glu-207 has been questioned, as it potentially could be sterically excluded by NAD and substrate binding [32] , [34] , this would for example not interfere with an activation of Cys-241 before substrate binding. It is also worth mentioning that the unusual positioning of NAD and the presumed pro- S stereoselectivity of ALDH3A1 (ref. 20 ) contributed to the hypothesis that Glu-268/399 (Glu-207/331 in FALDH) could have different functions in ALDH2 and ADLH3A1 (refs 34 , 36 ). Our finding of a similar stereoselectivity of FALDH and ALDH2 could therefore also point towards a comparable reaction mechanism. Substrate funnel properties and substrate specificity A distinctive structural feature in human FALDH is the presence of a novel structural element represented by an alpha helix (S446-L456) that directly follows the dimerization domain. This short helical segment extends over the substrate entry tunnel and originates from the adjacent subunit in the FALDH dimer ( Fig. 3 and Fig. 5d ). A short linker segment at the C-terminal end ( Fig. 2c ), connects the helix to the predicted transmembrane region (not present in the structural model). The novel helix is formed by a series of well-conserved residues in the FALDH protein family, most of which are hydrophobic (Val-448, Trp-450, Gly-451, Phe-453, Phe-454, Leu-455 and Leu-456; Figs 3a,b , 5a and Supplementary Fig. 5 ). The main axis of this helix forms a 90° kink with the preceding helix formed by amino acids 433–439 located at the edge of the substrate tunnel rim. As a consequence, helix 446–456 crosses over the tunnel entry. Both polar and hydrophobic interactions stabilize the configuration of helix 446–456. For example, the terminal amine group of Leu-447 (from the helix itself) forms a hydrogen bonding network with backbone atoms in a preceding loop region formed by amino acids 440–443 ( Fig. 5a ). Conversely, the side chain of Leu-455 at its C-terminal end inserts into a hydrophobic patch formed by the side chains of Leu-438 and Leu-89 at opposite sides of the rim. In this configuration, the helical segment closes the access to the cavity and very likely prevents the passage of substrates inside or outside the cavity. At the same time, a series of hydrophobic residues in this helical segment, including Trp-450 and Phe-453 as well as Phe-454 in the C-terminal linker region and Phe-459, form a prominent hydrophobic region oriented towards the outside over the substrate site and directed towards the presumed positions of the membrane ( Fig. 5a ). Interestingly, Leu-455 and Leu-456 in the helix and linker regions, respectively, are oriented towards the inner side of the cavity, restricting the available space on the upper part of the tunnel. This induces a 93° kink in the direction of the substrate cavity as calculated using the MOLE toolkit for PyMOL [42] . This configuration suggested that this unique C-terminal region might have an important ‘gatekeeper’ function, by controlling the access to the catalytic site and restricting the available space in the upper region of the substrate cavity. 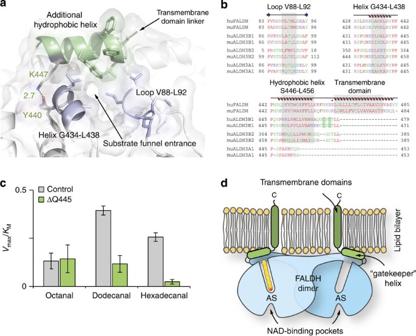Figure 5: Membrane interaction of FALDH. (a) A patch of hydrophobic amino acids (shown in stick model) is located around the FALDH substrate funnel entrance, originating from loop V88-L92, helix G434-L438 (both in lightblue) and the gatekeeper helix 446–456 in green. Correct orientation of the gatekeeper helix is supported by coordination of K447 to the backbone of Y440 (distance: 2.7 Å). The transmembrane domain linker indicates the position of the C-terminal transmembrane membrane domain. (b) Sequence alignment of human and mouse class 3 aldehyde dehydrogenase isozymes for loop V88-L92, helix G434-L438 and the gatekeeper helix S446-L456 (with Clustal Omega, see Methods). Residue colour scheme: hydrophobic, red; polar, green; charged (neg.), blue; charged (pos.), violet. Secondary structure was predicted with the human FALDH structure and the Stride software (http://webclu.bio.wzw.tum.de/stride/). Grey areas indicate (when present) corresponding regions in different isozymes. The introduced K463X stop codon in the FALDH expression construct is highlighted with a star. Cysteine residues in ALDH3B1 (indicated by green areas) represent lipidation sites for subsequent membrane anchoring. (c) Comparison of the catalytic capacity (Vmax/KM) of FALDH with (K463X) and without (Q445X) the gatekeeper helix to metabolize octanal, dodecanal and hexadecanal. No difference was found for octadecanal. With hexadecanal, theVmax/KMin Q445X was 10-fold lower (P=0.0003,t-test). Data are shown as mean±s.e.m. (calculated with error propagation,n=3). (d) Proposed model for FALDH membrane interaction. FALDH dimer is anchored into lipid bilayers via two transmenbrane domains. Hydrophobic patches (including the gatekeeper helix) around the substrate funnel reach into the membrane and allow efficient substrate (shown in yellow) turnover in the active site (AS). Positively charged residues around these patches increase membrane interaction (seeSupplementary Fig. 6a,b). NAD-binding pockets are directed away from the membrane and fully accessible. Figure 5: Membrane interaction of FALDH. ( a ) A patch of hydrophobic amino acids (shown in stick model) is located around the FALDH substrate funnel entrance, originating from loop V88-L92, helix G434-L438 (both in lightblue) and the gatekeeper helix 446–456 in green. Correct orientation of the gatekeeper helix is supported by coordination of K447 to the backbone of Y440 (distance: 2.7 Å). The transmembrane domain linker indicates the position of the C-terminal transmembrane membrane domain. ( b ) Sequence alignment of human and mouse class 3 aldehyde dehydrogenase isozymes for loop V88-L92, helix G434-L438 and the gatekeeper helix S446-L456 (with Clustal Omega, see Methods). Residue colour scheme: hydrophobic, red; polar, green; charged (neg. ), blue; charged (pos. ), violet. Secondary structure was predicted with the human FALDH structure and the Stride software ( http://webclu.bio.wzw.tum.de/stride/ ). Grey areas indicate (when present) corresponding regions in different isozymes. The introduced K463X stop codon in the FALDH expression construct is highlighted with a star. Cysteine residues in ALDH3B1 (indicated by green areas) represent lipidation sites for subsequent membrane anchoring. ( c ) Comparison of the catalytic capacity ( V max / K M ) of FALDH with (K463X) and without (Q445X) the gatekeeper helix to metabolize octanal, dodecanal and hexadecanal. No difference was found for octadecanal. With hexadecanal, the V max / K M in Q445X was 10-fold lower ( P =0.0003, t -test). Data are shown as mean±s.e.m. (calculated with error propagation, n =3). ( d ) Proposed model for FALDH membrane interaction. FALDH dimer is anchored into lipid bilayers via two transmenbrane domains. Hydrophobic patches (including the gatekeeper helix) around the substrate funnel reach into the membrane and allow efficient substrate (shown in yellow) turnover in the active site (AS). Positively charged residues around these patches increase membrane interaction (see Supplementary Fig. 6a,b ). NAD-binding pockets are directed away from the membrane and fully accessible. Full size image To test this hypothesis, we removed the gatekeeper helix in FALDH by introducing an early stop codon at position Gln-445 and compared its capacity with metabolized aldehyde substrates with differing chain lengths. We found that in these mutants, the V max / K M ratio for the medium chain aldehyde octanal is not altered (C 8 ), indicating that this mutation does not compromise the catalytic capacity. Remarkably, however, when the longer fatty aldehydes docecanal (C 12 ) and hexadecanal (C 16 ) were used as substrates, the absence of the gatekeeper helix resulted in a substantially lower catalytic capacity (threefold and tenfold lower, respectively; Fig. 5c ). Notably, a mutation in this structural element (K447E) is reported to cause SLS [43] . Lys-447 is located at the gatekeeper helix and in the present structure is engaged in a hydrogen bond network that stabilizes the closed conformation ( Fig. 5a ). Together, these data indicate that the gatekeeper helix of FALDH does not participate directly in catalysis, but is required for the efficient turnover of long-chain fatty aldehydes. The gatekeeper helix represents a unique structural feature compared with the more accessible and linear substrate funnel found in ALDH3A1 ( Fig. 5c ), which completely lacks this structural component. FALDH membrane interaction Two transmembrane domains anchor the FALDH dimer to membranes (Scheme in Fig. 5d , dark green). These transmembrane helices, which were not present in our expression constructs, starts four amino acids after Asn-460, the last residue with well-defined electron density in the proposed FALDH structure. This implies that—once the transmembrane helices are inserted in the lipid bilayer—the two substrate funnel entries and their respective gatekeeper helices would be oriented towards the lipid bilayer, while the cofactor binding pockets would be both directed towards the cytosolic side ( Fig. 5d ). Interestingly, a series of surface-exposed side chains form a hydrophobic ring around the substrate funnel entrance oriented towards the membrane ( Fig. 5a , hydrophobic residues shown in stick model). These residues originate from the gatekeeper helix itself (Val-448, Trp-450, Phe-453, Phe-454, Leu-455, Leu-456; Fig. 5a , green), from loop V88-L92 (Val-88, Leu-89, Met-91, Leu-92; Fig. 5a , blue) and from the 3 10 -helix G434-L438 (Ala-435, Leu-438; Fig. 5a , blue). The hydrophobic patches could allow the FALDH substrate-binding funnels to reach into membranes in order to facilitate efficient substrate binding. Moreover, the hydrophobic patches are surrounded by positively charged residues (Lys-85, Lys-431, Arg-432 and Arg-436), which can interact with the negatively charged head groups of the lipid bilayer ( Supplementary Fig. 6a,b ) and are conserved in the FALDH protein family ( Fig. 5b , Supplementary Figs 2,5 ). Molecular mechanism of SLS-causing mutations Using the novel structural information, we investigated the molecular mechanism of missense mutations known to cause SLS. We classified the mutations according to their expected effects on the active site ( Fig. 6 , red), dimerization ( Fig. 6 , green), protein misfolding ( Fig. 6 , orange) and special mutations ( Fig. 6 , blue). The effect on protein stability was estimated by calculating ΔΔ G values with the empirical FoldX force field (Methods). A detailed list of all mutations can be found in Supplementary Table 1 . 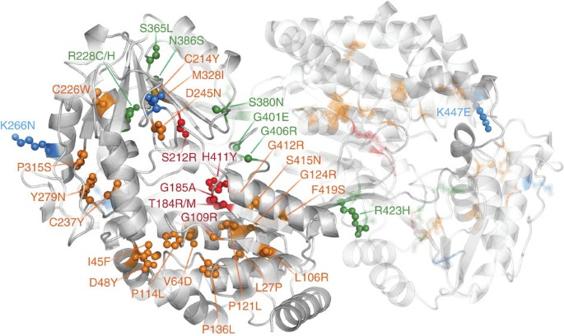Figure 6: Point mutations causative for the SLS and affected residues in the FALDH structure. The FALDH backbone is shown in white cartoon representation. Residues affected by SLS-causing mutations are shown in ball and stick representation and were coloured according to the assumed molecular implication. Orange, mutations leading to protein misfolding (19). Green, mutations at the dimerization interface (8). Red, mutations affecting the catalytic site (5). Blue, special mutations (3). For a detailed list, seeSupplementary Table 1. Figure 6: Point mutations causative for the SLS and affected residues in the FALDH structure. The FALDH backbone is shown in white cartoon representation. Residues affected by SLS-causing mutations are shown in ball and stick representation and were coloured according to the assumed molecular implication. Orange, mutations leading to protein misfolding (19). Green, mutations at the dimerization interface (8). Red, mutations affecting the catalytic site (5). Blue, special mutations (3). For a detailed list, see Supplementary Table 1 . Full size image The structure of human FALDH presented here reveals a novel structural element at its C-terminal region that controls access to the substrate cavity and plays an important role in the discrimination towards long-chain fatty aldehydes. This novel structural feature is conserved in other membrane-associated dehydrogenases and helps explain the phenotype of a number of mutations associated with SLS. FALDH adopts a dimeric structure ( Fig. 2 ), similar to soluble ALDHs [14] , [16] , [20] , especially to the closely related ALDH3A1. However, a distinctive feature of FALDH is the presence of a hydrophobic helix and a single transmembrane helix that follows directly after the oligomerization domain. The hydrophobic helix is evolutionary conserved across species ( Supplementary Fig. 5 ). In this structure, the hydrophobic helix covers the substrate tunnel entry, acting like a cap or gatekeeper ( Fig. 3a ). Removal of this gatekeeper helix in the truncated Q445X version of FALDH strongly reduced the catalytic capacity of the enzyme towards hexadecanal, but not towards the shorter-chained octanal ( Fig. 5c ). The SLS-associated single missense mutation K447E [43] indicates that the gatekeeper helix also plays an important role in the development of SLS. Lys-447 originates from the gatekeeper helix and forms a hydrogen bond with the peptide backbone of Tyr-440 ( Fig. 5a ), thereby contributing to stabilize the gatekeeper helix in the closed conformation. The mechanism through which the gatekeeper helix confers higher efficiency towards long-chain substrates is not completely clear. One possibility is that the helix is required to facilitate transit of substrates and products between membranes and the substrate cavity. At the same time, side chains from the inner side of the helix are oriented towards the inside of the cavity, which introduces a change in direction of the substrate tunnel and constrains the space available at the upper section of the tunnel ( Fig. 3a ). Consequently, fatty aldehydes fitting to the modified geometry of the FALDH substrate funnel have to display a certain degree of flexibility in their hydrophobic carbon chains. Moreover, the closed conformation of the gatekeeper helix may restrict the conformation of substrate molecules within the cavity, which can be important to productively orient the polar head of the substrate within the catalytic site. Side chains from amino acids lining the substrate channel itself are also likely to participate in substrate selection. The width of the FALDH tunnel would allow only a limited number of branching side methyl groups, but does not seem compatible with larger aromatic, mainly unsaturated or strongly branched molecules. Together, these factors are likely to contribute in shaping the substrate specificity of FALDH and could explain why the rigid, polyunsaturated fatty aldehydes all-trans-retinal and 11-cis-retinal have not been reported as substrate for FALDH [44] . In addition to the membrane insertion and orientation via two C-terminal transmembrane domains, the gatekeeper helix and the hydrophobic loops V88-L92 and G434-L438, the presence of positively charged amino acids surrounding the patch of hydrophobic residues around the gatekeeper helix might facilitate interaction with phospholipid head groups at the membrane ( Supplementary Fig. 6b ). Comparable configurations of hydrophobic and positively charged residues have been found in in other membrane-associated enzymes, like cyclooxygenases [45] and could provide a molecular basis to understand how long-chain lipids transit from the membrane to the substrate cavities. Analysis of class 3 ALDHs suggests that the gatekeeper helix may be a distinctive feature of membrane-associated enzymes. For example, ALDH3B1 is a membrane-associated ALDH, and multiple sequence alignments ( Fig. 5b , grey areas) show that it also contains a region with helical propensity and rich hydrophobic residues in a region equivalent to that of the FALDH gatekeeper helix ( Fig. 5b ). In contrast, ALDH3B1 has no transmembrane helices. Instead, this enzyme is anchored to plasma membranes via C-terminal palmitoylation and prenylation (lipidated cysteines are marked in green, Fig. 5b ) (ref. 46 ). Membrane insertion through lipid modification in this enzyme would result in a configuration similar to that of FALDH ( Fig. 5d ). Interestingly, biochemical experiments revealed that the substrate specificity of ALDH3B1 resembles FALDH [46] , [47] and that it also participates in protection against lipid-derived oxidative stress [48] , [49] . However, in contrast to FALDH, ALDH3B1 has no implication in sphingosine-1-phosphate metabolism [46] , which is in agreement with studies that show the sphingosine-1-phosphate producing Sphingosine-1-phosphate lyase localizes, analogue to FALDH, in the endoplasmic reticulum [50] . Our results indicate that, although membrane anchoring of FALDH and ALDH3B1 is achieved in two different ways, both enzymes could facilitate their specificity towards long-chain fatty aldehydes by the same molecular interaction of their hydrophobic patches with the lipid bilayer. The conservation of these respective regions can also be found in ALDH3B2 ( Fig. 5b ), an enzyme closely related to ALDH3B1, which has so far not been studied in detail. In contrast, ALDH3A1 is a cytosolic enzyme that processes more soluble aldehydes and functions in the protection of corneal crystalline against UV-light-induced damage [51] . Although ALDH3A1 is the closest aldehyde dehydrogenase to FALDH in terms of overall sequence conservation (66% sequence identity), it completely lacks the hydrophobic regions corresponding to the gatekeeper helix ( Fig. 5b ) [14] . Moreover, ALDH3A1 also lacks the additional hydrophobic domains in loops the V88-L92 and G434-L438 that together with the gatekeeper helix form the hydrophobic ring around the substrate tunnel entry ( Fig. 5b ). This indicates that these features are specific adaptations of membrane-associated ALDHs. In other class 1 and 2 ALDHs, an equivalent for G434-L438 and the gatekeeper helix is completely missing (sequence alignment of all class 1–3 ALDHs in Supplementary Fig. 2 ). Rizzo et al . [4] reviewed 72 different mutations of the ALDH3A2 gene associated with SLS. Since then a series of novel mutations have been reported [52] , [53] , [54] , [55] , [56] , [57] , [58] , [59] , [60] , [61] , [62] , [63] . These include missense mutations (40.9%), deletions (25%), splice site mutations (13.6%), insertion (10.2%), nonsense mutations (6.8%) and some complex mutations (4.5%), which are likely to compromise production of the active FALDH protein. However, a considerable proportion (40.9%) of SLS-associated alleles carries missense mutations leading to single amino-acid substitutions. The structural and biochemical analysis presented here provides a basis to understand the molecular mechanisms underlying the disease in these patients. We classified the group of missense mutations into four categories according to their expected effects ( Fig. 6 ). A first group corresponds to mutations that are likely to destabilize the FALDH protein fold through various mechanisms. This includes for example, the introduction or substitution of proline residues at critical positions (L27P, P114L, P121L, P136L, P315S), or the modification of either the polarity or the size of side chains located at the hydrophobic core of the protein (D48Y, V65D, L106R, G124R, D245N, F419S, I45F, C214Y, C226W, C237Y, Y279N, S415N, C421R; Fig. 6 , orange). These mutations are likely to lead to reduced FALDH function by inducing misfolding and/or increased proteolytic degradation. Another group of missense mutations (five mutations) involve residues at, or in the vicinity of the active and cofactor binding sites and likely to compromise catalytic activity ( Fig. 6 , red). A summary of all missense mutations and a quantitative estimation of protein fold stability can be found in Supplementary Table 1 . A series of mutations with previously elusive aetiology involves residues at the dimerization interface and the gatekeeper helix ( Fig. 6 , green). In an earlier work, we could show that native FALDH is active as a dimer [18] . The present work reveals that the gatekeeper helix plays a critical role in the function of FALDH and that dimerization is required both to position this helix over the substrate tunnel of the adjacent subunit and to orient the two catalytic sites towards the lipid bilayer. In agreement with this, a naturally occurring mutation that completely removes the transmembrane domain together with the gatekeeper helix (premature stop codon: K437X) has been reported to cause SLS [62] . Other illustrative examples are the gatekeeper helix mutation K447E (discussed above) or mutations involving residues Ser-380 and Arg-423 at the dimerization interface (SLS mutations S380N or R423H). These residues form two reciprocal interaction pairs across the dimer interface. Mutation of either one or the other residue would result in loss of critical hydrogen bonds at two symmetric sites of the dimerization interface leading to a significant destabilization of the dimer. Finally, the mutation K266N has been shown to cause instability of the mRNA [43] . The structure of FALDH shows that Lys-266 lies on the surface of the protein at a region relatively distant to the cofactor, catalytic or substrate tunnel sites. The Lys-266 residue’s side chain is oriented towards the solvent and does not seem to be directly involved in interactions with other residues. Hence, the reported effect in mRNA stability rather than a potential effect on protein structure and stability appears the most likely explanation of how the K266N mutation causes the SLS. We also investigated if the characteristic substrate specificity of FALDH towards longer chained aliphatic aldehydes is reflected by changes within the catalytic center, which was of particular interest given the uncommon catalytic mechanism (based on a FALDH homology model with the structure of rat ALDH3A1) that had been suggested previously [19] . However, the findings presented herein support a reaction mechanism, that closely resembles the mechanisms previously reported for other members from the ALDH superfamily ( Fig. 4a ). A special NAD-binding mode for ALDH3A1 has been reported [14] , [20] , [32] , which was discussed to point towards a pro- S instead of a pro- R specificity of class 3 ALDHs [20] . However, our experimental results indicate unambiguously a pro- R specific mode for hydride transfer during catalysis ( Fig. 4c ), similar to that of class 1 and 2ALDH isozymes. This is also in agreement with a pro- R specific binding mode of NAD found in a recent structure of ALDH3A1 (ref. 21 ) and with a consistent pro- R stereospecificity measured in different ALDHs, including native plasma-encoded hepatic tumor-associated aldehyde dehydrogenase, which by detailed biochemical analysis was identical to ALDH3A1 (ref. 23 ). The data presented here suggest that membrane-associated ALDHs achieve their specific physiological role in detoxifying lipophilic aldehydes through specialized structural elements at the interface between the lipid bilayer and their substrate cavity in combination with their tissue and cell type specific expression patterns [13] , [18] . The newly identified gatekeeper region is essential to understand how this enzyme facilitates its cellular function and provides a mechanistic rationale for a series of mutations causing the SLS. Cloning and site-directed mutagenesis Human FALDH cDNA was obtained from Imagenes (Berlin, Germany). The human FALDH insert was then subcloned with BamHI/SacII into the pPR-IBA2 Strep-tag fusion vector (IBA, Goettingen, Germany) (see Supplementary Table 2 for primers). This vector allowed expression of FALDH in E.coli in fusion with a single N-terminal strep-tag. Twelve amino acids were introduced between the strep-tag sequence and the first methionine of FALDH. To increase solubility of FALDH an early stop codon was introduced near the C terminus of the enzyme, removing the 22 amino acids of transmembrane helix, by site-directed mutagenesis into huFALDH_pPR-IBA2 vector using appropriate primers (K463X, see supplementary Table 2 ) and the QuikChange Site-Directed Mutagenesis kit (Stratagene). Mutants N112A, Y113F, E207Q, C241S, E331Q, Y410F and Q445X were generated similarly by site-directed mutagenesis (primers see supplementary Table 2 ). Correct integration of all constructs was verified by sequence analysis (Microsynth, Balgach, Switzerland). Expression and purification pPR-IBA2 plasmids containing either wild-type or mutated versions of FALDH were transformed into Single Step (KRX) Competent Cells (Promega). FALDH activity was measured at different points of the purification using the fluorescence labelled fatty aldehyde pyrenedecanal (Rambius, Lund, Sweden) as described in [18] . Briefly, samples were incubated for 10 min at 37 °C with 25 mM sodium pyrophosphate pH 8.0, 0.1% Triton X-100 and 1 mM NAD and 50 μM pyrenedecanal as substrate in a total volume of 10 μl. Reactions were stopped by addition of 30 μl of methanol. After centrifugation, 10 μl of the supernatant was injected on an Agilent 1200 Series HPLC system using a Zorbax XDB-C8 USP-L7 column (Agilent Technologies, Vienna, Austria). Elution of fluorescence labelled substrate and product was monitored with fluorescence detection (excitation: 340 nm; emission: 400 nm). Peak areas were quantified with external calibration using pyrenedecanoic acid (Sigma) as standard. KRX cells were grown in TB-medium at 37 °C until they reached OD 600 =1.0 and were then induced with L-rhamnose/Isopropyl-β-D-1-thiogalactopyranoside (0.1% (w/v)/1 mM). After further incubation at 25 °C for 24 h, the bacterial pellets were collected, resuspended in buffer (100 mM potassium phosphate, pH 7.5, 1 mM DTT, 1 mM EDTA), treated with 0.2 mg ml −1 lysozyme (total volume of 20 ml per liter TB-medium) in for 15 min at 25 °C and subsequently lysed in a French press (Aminco, SLM Instruments, Rochester, USA). Insoluble components were removed by centrifugation (30 min 4 °C, 45,000 g ). The supernatant was loaded on a Strep-Tag affinity column (IBA, Goettingen, Germany). The bound protein was eluted with D-desthiobiotin (IBA), concentrated and washed with 50 mM triethanolamine pH 7.0 in spin filtration units (10 kDa Amicon Ultra, Millipore, Vienna, Austria). The sample was then subjected to gel filtration with a Superose 12 10/300 GL column (Tricon, 17‐5173‐01) using 50 mM triethanolamine, 150 mM NaCl pH 7.0 as buffer. Fractions containing FALDH were concentrated and washed again in spin filtration units (5 kDa, Millipore), flash-frozen in liquid nitrogen and subsequently stored at −80 °C at a concentration of 15.5–17.7 mg ml −1 in 50 mM triethanolamine pH 7.0 containing 150 mM NaCl. Protein purity was checked by SDS-page with Coomassie staining and correct protein folding was validated by circular dichroism measurements. Crystallization, data collection and structure solution The FALDH protein was assayed for crystallization High Throughput Crystallization Laboratory of the EMBL Grenoble Outstation ( https://embl.fr/htxlab ) by the vapour diffusion method [64] . Single three-dimensional crystals were obtained by mixing 100 nl of protein solution at a concentration of 15 mg ml −1 and 100 nl of crystallization solution (0.2 M Li 2 SO 4 , 0.1 M CHES pH9.5, 1.0 M K/Na tartrate). Crystals were transferred to a solution containing crystallization solution supplemented with 15% glycerol and cryo-cooled in liquid nitrogen. The FALDH crystals belonged to space group P 2 1 2 1 2 1 and diffracted up to a resolution of 2.1 Å. X-ray diffraction experiments were performed at the beamline PROXIMA1 of the synchrotron SOLEIL and the MX beam lines of the European Synchrotron Radiation Facility (ESRF). Crystallographic data reduction and scaling was carried out with the software XDS [65] . Initial phases were obtained by the molecular replacement method using Phaser [66] and the atomic coordinates of the human ALDH3A1 protein (3SZA) [16] as search model. Successive rounds of automatic refinement and manual building were carried out with RefMac5 (ref. 67 ) and Coot [68] . Illustrations were produced with Pymol ( http://www.pymol.org ) and MOLE [42] . Multiple Sequence Alignment of FALDH and ALDH3A1 from different species were calculated with the Clustal Omega ( http://www.ebi.ac.uk/ ) and the following sequences: CAG33703.1, NP_031463.2, NP_113919.2, AAI49985.1, NP_001128640.1, NP_114178.1, NP_001159985.1. Measurement of FALDH activity Kinetic constants of FALDH wild type and mutants were determined with a Fluoroskan Ascent Microplate Reader (Thermo Fisher Scientific, Vienna, Austria) via the conversion of cofactor NAD to NADH, which was followed fluorometrically (excitation: 355 nm; emission: 460 nm). Reactions were carried out at 37 °C in 96-well plates in a buffer containing 25 mM sodium pyrophosphate pH 8.0, 0.1% Triton X-100 and 1 mM NAD. Octadecanal (Sigma), dodecanal (Sigma) and hexadecanal were used as substrates. Hexadecanal was a generous gift of Dr Karsten Lange (Organic Chemistry Department, Bergische Universität Wuppertal, Germany) and was synthesized as described in Isopropyl-β-D-thiogalactopyranoside (ref. 22 ). Briefly, n-Hexadecanol (in dry CH 2 Cl 2 ) was placed on ice and treated with dry DMSO and P 2 O 5 . After stirring for 2 h at room temperature, the mixture was cooled down to 0 °C and triethylamine was added dropwise, followed by stirring at room temperature for 1 h. The reactions mixture was mixed with water and the pH adjusted to pH=2 with HCl. After phase separation, the organic layer was collected, dried and purified via short column chromatography. Product quality was confirmed by 1 H- and 13 C-NMR. Substrates were used as in nine dilutions in the range of 0.005–300 μM. K m and V max values were determined by using NAD at saturating concentrations and varying the concentrations of substrates between 0 and 300 μM. The reaction was started by the addition of protein and was followed for 120 min with one measurement point per minute. Reaction rates were determined via the slope within the linear range of the resulting curves and calibrated with external NADH dilution series. Statistical analysis to determine K m and V max was done by fitting reaction rate and concentration data with the Michaelis Menten analysis package implemented in GraphPad Prism (GraphPad Software Inc., La Jolla, USA). Determination of stereospecificity through NMR and ESI-MS The stereospecificity of the hydride transfer was investigated by NMR spectroscopy on a Bruker 600 MHz Avance II+ instrument. The enzymatic reaction was performed in total volume of 500 μl in a standard 5 mm NMR tube and was monitored in real time. All reaction components (25 mM sodium pyrophosphate, 1 mM NAD, 300 μM isotope labelled 1-[D]-hexadecanal (Tocris Bioscience, Bristol, United Kingdom) from a 50-fold stock in ethanol) and 10% D 2 O were premixed in the NMR tube and equilibrated at 37 °C in the NMR spectrometer followed by a shimming procedure. Then, the tube was removed from the spectrometer and the enzymatic reaction was initiated by the addition of 3.5 μg purified FALDH in a minimal volume (2.5 μl) without changing the position of the tube in the spinner. Without further shimming procedures to minimize the dead time the reaction was followed via a series of 1D– 1 H NMR spectra acquired in a pseudo-2D manner. As a control, we analysed the reaction of 1,2-[D]-ethanol (Sigma) and alcohol dehydrogenase equine (with known pro- R stereosectivity, 79854, Sigma) under the same conditions. The direct hydride transfer was also verified on a Finnigan MAT 95S mass spectrometer operated in positive ESI ionization-mode at a spray voltage of 1.4 kV. Enzymatic reaction was carried out under the same conditions except for using 20 mM Triethanolamine pH 8.0 as buffer. Reactions were stopped after 10–300 min by addition of a threefold excess of methanol and the reaction mixture was directly injected into the mass spectrometer. Quantitative estimation FALDH protein fold stability Differences in fold stability of wild-type and mutated FALDH was estimated using empirical FoldX force field version 3.0 allowing for quantitative estimation of differences in protein fold stability [69] , [70] . After a relaxation of the structure in the FoldX force field using ‘repairpdb’, in silico mutations were calculated allowing neighbouring residues to rearrange. To test robustness of FoldX predictions, we performed five individual runs for each of the two subunits of FALDH, leading to 10 individual estimations per mutation. Water molecules resolved in the crystal structure were retained in calculations, the ionic strength of the surrounding solution was set to default 0.050 M. Temperature was set to 298 K, the pH to 7.0. How to cite this article: Keller, M. A. et al . A gatekeeper helix determines substrate specificity of Sjögren–Larsson Syndrome enzyme fatty aldehyde dehydrogenase. Nat. Commun. 5:4439 doi: 10.1038/ncomms5439 (2014). Accession codes: The atomic coordinates and structure factors corresponding to the structure presented in this work have been deposited in the Protein Structure Databank (PDB) under the accession code 4QGK .